Evolutionary-guidedde novostructure prediction of self-associated transmembrane helical proteins with near-atomic accuracy How specific protein associations regulate the function of membrane receptors remains poorly understood. Conformational flexibility currently hinders the structure determination of several classes of membrane receptors and associated oligomers. Here we develop EFDOCK-TM, a general method to predict self-associated transmembrane protein helical (TMH) structures from sequence guided by co-evolutionary information. We show that accurate intermolecular contacts can be identified using a combination of protein sequence covariation and TMH binding surfaces predicted from sequence. When applied to diverse TMH oligomers, including receptors characterized in multiple conformational and functional states, the method reaches unprecedented near-atomic accuracy for most targets. Blind predictions of structurally uncharacterized receptor tyrosine kinase TMH oligomers provide a plausible hypothesis on the molecular mechanisms of disease-associated point mutations and binding surfaces for the rational design of selective inhibitors. The method sets the stage for uncovering novel determinants of molecular recognition and signalling in single-spanning eukaryotic membrane receptors. Protein associations regulate the function of a large diversity of membrane proteins, such as tyrosine kinase (RTK), cytokine, immune or G protein-coupled receptors [1] , [2] , [3] , [4] , [5] . Single spanning receptors such as RTKs can adopt multiple conformations and function by extracellular ligand-induced stabilization of specific receptor homo- or heterodimeric conformations triggering activation of cytoplasmic signalling cascades [6] , [7] , [8] , [9] . By changing orientation or oligomerization states, transmembrane (TM) and juxtamembrane (JM) regions play critical roles in regulating receptor associations and in transmitting signals across the membrane [7] , [8] , [10] . Numerous point mutations in their TM or TM–JM boundary regions perturb the receptor’s conformations and functions, and are associated with severe disease [1] , [11] , [12] , hence the importance of determining their structure for rational drug design applications. However, compared with multi-pass membrane proteins, single-pass oligomeric membrane receptors (SPMRs) are highly flexible and remain very difficult to characterize structurally. Several extramembrane (EM) and a few TM domains have been characterized by X-ray crystallography and nuclear magnetic resonance (NMR) spectroscopy [13] , [14] , [15] , [16] , [17] , [18] , respectively, but no high-resolution structure of a full-length SPMR has been solved to date. Nevertheless, current evidence on widely studied receptors such as epidermal growth factor receptor (EGFR) and integrin indicate that TM interactions and structures determined from isolated domains are consistent with those in full-length receptors [8] , [9] , [19] , [20] , [21] . Thus, the structural characterization of isolated TM domains can be considered as a valid first approach to identify native TM–TM interactions in full-length receptors. When extensive experimental information is available on TM interactions (for example, mutational, crosslinking, infrared spectroscopy and homologue structures), TM structures can be modelled accurately [22] and full-length receptor structures can be reconstructed by linking EM structures with TM models [19] . However, such experimental information is not available for a large majority of SPMR TMs, which can only be modelled from sequence. The first characterized TM homodimer structures were of right-handed conformations and stabilized by the frequently occurring GXXXG-binding motif through putative weak CαH–O hydrogen bonds [15] . Corroborating these observations, modelling techniques incorporating a weak CαH–O bond potential allowed for accurately predicting native right-handed TMH homodimer (RH) structures in native TMH docking simulation [23] or grid search from ideal helices [24] . However, a large majority of TMH homo-oligomers does not bear GASright motifs (that is, small-XXX-small residue motif identified at right-handed parallel TMH dimers with small being either Gly, alanine or serine [25] ) or are stabilized by a much larger diversity of physical interactions including Van der Waals (VDW), aromatic pi–pi, cation–pi and polar interactions [3] , [6] , [26] , [27] , [28] , [29] . Accurately predicting TMH oligomeric structures in absence of monomer TMH structures and of specific binding motifs identifiable from the sequence remains a daunting task, because of the large conformational space to be sampled in simultaneously folding and docking TMHs. Approximating TMHs as ideal helices usually cannot recapitulate TM dimer structures with near-atomic accuracy [30] . As demonstrated by several studies [31] , [32] , [33] , [34] , because protein interactions are very sensitive to atomic details, designing selective inhibitors and predicting functional mechanism or mutational effects require high-resolution models (that is, typically structural divergence to native structures below 1.5 Å and a large fraction of predicted native contacts). A general method that predicts with high accuracy from sequence the structure of TMH oligomers with a wide range of TMH subunits, topologies, conformations and stabilizing interactions would therefore be of great interest but is currently lacking. Rapid expansion of high-throughput sequencing and statistical methods distinguishing direct couplings from indirect correlations in residue sequence covariation patterns have led to high-precision residue contact prediction in protein structures [35] , [36] , [37] , [38] , [39] , [40] , [41] . Applying these predicted contacts as distance constraints in folding simulations considerably restrict the conformational space sampled and allowed for the reliable prediction of large polypeptide chain structures [42] , [43] . Co-evolutionary-based protein modelling approaches have recently been extended towards characterizing protein conformational diversity including the structure of transient or hidden functional states [44] . Residue contacts controlling important functional protein–protein interactions can also be identified in sequence co-evolution patterns of strongly interacting proteins [45] , [46] . When combined with protein surface chemical complementarities, such contacts can guide the prediction of both stable and transient protein–protein-associated structures [47] . However, applying this approach to homo-oligomers remains a challenge, because it relies on the ability to discriminate between intra- and inter-monomer contacts. To address this problem, we here develop and implement in RosettaMembrane [23] , [34] , [48] EFDOCK-TM (Evolutionary-guided Fold and Dock of TransMembrane proteins), a protocol to accurately predict self-associated TM protein structures guided by co-evolutionary signals enriched in true inter-chain contacts using predicted TMH binding surfaces from sequence. We show that a very small number (less than three on average) of these selected contacts are necessary to accurately predict single-spanning TMH homo-oligomer structures with a wide range of size, subunit number, conformations and binding interactions. We apply EFDOCK-TM to blindly predict uncharacterized members of the KIT and fibroblast growth factor receptor (FGFR) family of RTK receptors and propose molecular interpretations of disease-occurring point mutations. Inter-chain-contacting residues co-evolve strongly The structural interpretation of co-evolutionary signals in protein sequences folding into homo-oligomers has been a challenge, because they can in principle reflect both intra-chain and inter-chain residue contacts. When sequences fold into parallel helical homo-oligomers, discriminating between intra- and inter-monomer constraints becomes even more difficult because both encode short-range contacts (that is, between residues close in sequence) ( Fig. 1a ). We define a short-range intra-chain contact, an interaction between residues i and j close in sequence and on the same monomer chain A (i A —j A ≤8). We define a short-range inter-chain contact, any interaction between residues i and j close in sequence but belonging to distinct chains A and A′ in a homodimer formed by two copies of the same monomer sequence (i A —j A′ ≤8) ( Fig. 1a ). Since most residues in helices are involved in short-range intra-chain contacts, we reasoned that the fraction of residue pairs forming additional inter-chain short-range interactions should be enriched in strongly co-evolving residues at the binding interface ( Fig. 1b ). To test this hypothesis, we first analysed the strength of residue covariations along the binding interface of all experimentally characterized TMH homodimer structures. Residue covariations were calculated using the widely used and benchmarked method EVfold [42] . As shown in Fig. 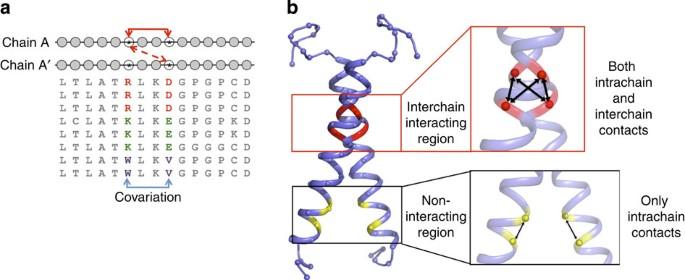Figure 1: Covariation in protein sequences folding as homo-oligomers reflect both intra- and inter-molecular contacts. (a) Covariation patterns in protein sequences forming homo-oligomeric structures can reflect both intra- (solid red arrow) and inter- (dash red arrow) monomer evolutionary constraints. (b) The strength of co-evolution signals between residues forming both intra- and inter-chain contacts (red) is expected to be stronger (thicker arrows) than pairs forming only intra-chain contacts (yellow, thinner arrows at the bottom). 2a,b and Supplementary Table 1 , the average direct interaction (DI) score (measuring the strength of co-evolution) and the fraction of strongly co-evolving residues (high DI score) calculated by EVfold were significantly higher for residue pairs involved in inter-chain contacts than for other residues present at the binding interface. Similar results were obtained when the same analysis was performed on a large data set of coiled-coil homodimers selected from diverse protein families (Methods; Supplementary Table 1 ). These results validate our hypothesis and indicate that co-evolutionary signals at homodimer helical binding interfaces are often stronger for residue pairs involved in inter-chain contacts than for pairs forming intra-chain contacts only. Figure 1: Covariation in protein sequences folding as homo-oligomers reflect both intra- and inter-molecular contacts. ( a ) Covariation patterns in protein sequences forming homo-oligomeric structures can reflect both intra- (solid red arrow) and inter- (dash red arrow) monomer evolutionary constraints. ( b ) The strength of co-evolution signals between residues forming both intra- and inter-chain contacts (red) is expected to be stronger (thicker arrows) than pairs forming only intra-chain contacts (yellow, thinner arrows at the bottom). 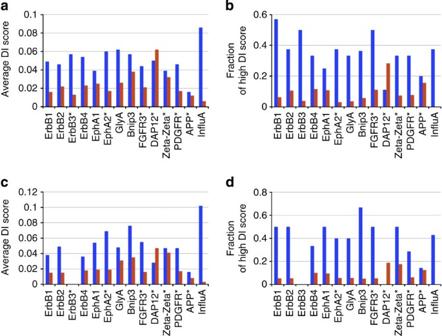Figure 2: Residue pairs making inter-chain contacts have stronger co-evolutionary signals. Comparison between direct interaction score (DI score) calculated by EVfold42for residue pairs interacting (blue) or not interacting (red) across the chains of the 14 TM homo-oligomers indicated on thexaxis. Only short-range residue pairs (that is, separated by up to eight amino acids) that belong to either the true binding interface (a,b) or the predicted binding helical surface by LIPS49(c,d) are considered in the analysis (Methods). The average DI score for all residue pairs (a,c) or the percentage of high DI score pairs (b,d) in each interacting category is reported (Methods). DI score differences between the two populations of residue pairs are statistically significant (paired two-sampleT-testPvalues <4 ×E−03, seeSupplementary Fig. 2). Full size image Figure 2: Residue pairs making inter-chain contacts have stronger co-evolutionary signals. Comparison between direct interaction score (DI score) calculated by EVfold [42] for residue pairs interacting (blue) or not interacting (red) across the chains of the 14 TM homo-oligomers indicated on the x axis. Only short-range residue pairs (that is, separated by up to eight amino acids) that belong to either the true binding interface ( a , b ) or the predicted binding helical surface by LIPS [49] ( c , d ) are considered in the analysis (Methods). The average DI score for all residue pairs ( a , c ) or the percentage of high DI score pairs ( b , d ) in each interacting category is reported (Methods). DI score differences between the two populations of residue pairs are statistically significant (paired two-sample T -test P values <4 × E −03, see Supplementary Fig. 2 ). Full size image Most single-spanning self-associating receptors, however, are largely uncharacterized with no information on their binding interfaces. To address this problem, we assessed whether TMH-interacting surfaces could be predicted from sequence by the method LIPid-facing Surface (LIPS) [49] . On average, 85% of the residues predicted by LIPS to be the least exposed to lipids were located at the experimentally characterized binding interface ( Supplementary Fig. 1 ). As shown in Fig. 2c,d , when combined with the method EVfold, the method LIPS [49] was able to predict from sequence TMH surfaces that bear a large fraction of strongly co-evolving contacts. Both average DI score and fraction of strongly co-evolving contacts were found to be significantly higher for residues predicted to interact across monomers than for other residues along the predicted binding interface ( Supplementary Table 1 ). Our results indicate that the prediction of interacting TMH surfaces by LIPS is accurate enough to identify a large majority of the strongly co-evolving residue pairs involved in inter-chain contacts. Enrichment of intermolecular contacts in blind predictions To take advantage of such signals in blind prediction of TMH homomeric structures, we implemented a computational framework that enriches co-evolving residue pairs in true inter-chain contacts ( Fig. 3 ). Briefly, (1) contacts between pairs of co-evolving residues along the entire TM region are predicted from sequence using the method EVfold [42] ; (2) contacting residues present on TMH surfaces predicted to face lipids using the method LIPS [49] are removed; (3) the remaining contacts with the strongest co-evolutionary signals, which are often enriched in inter-chain contacts ( Fig. 2 ), are selected as pairwise distance constraints; (4) simulations using EFDOCK-TM, a protocol that we developed in this study and implemented within RosettaMembrane [23] , [34] , [48] for folding and docking TMH oligomers (Methods) are performed in parallel with randomly selected subsets of constraints until all possible combinations of constraints are enumerated. Representative low-energy models of TMH homo-oligomers were selected from the best converged simulations generating the least clusters (Methods). 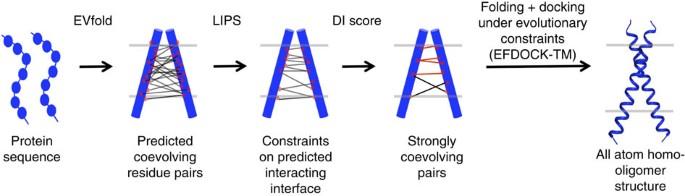Figure 3: Evolutionary-guidedde novostructure prediction of TMH homo-oligomer using EFDOCK-TM. Stepwise selection of inter-chain contacts and structural models. Step 1: EVfold—this method42is used to predict co-evolving residue pairs likely in physical contacts in the protein structure (black lines). Step 2: LIPS—this method49is used to predict the helical surface that has the highest propensity to self-associate. Predicted contacts which do not belong to this surface are filtered out. Step 3: DI score—predicted contacts with low co-evolutionary DI scores are filtered out (true interacting sites are depicted in red, and false interacting sites are in black). Step 4: Convergence and energy-guided selection of models—folding and docking EFDOCK-TM simulations enumerating all possible combinations of constraints defined by subsets of predicted contacts are performed, leading to different levels of convergence. A total of 10,000 trajectories and final models are generated per simulation. Representative models are selected among the centres of the five largest families obtained by clustering the 10% lowest-energy models generated by the most-converged simulation. Figure 3: Evolutionary-guided de novo structure prediction of TMH homo-oligomer using EFDOCK-TM. Stepwise selection of inter-chain contacts and structural models. Step 1: EVfold—this method [42] is used to predict co-evolving residue pairs likely in physical contacts in the protein structure (black lines). Step 2: LIPS—this method [49] is used to predict the helical surface that has the highest propensity to self-associate. Predicted contacts which do not belong to this surface are filtered out. Step 3: DI score—predicted contacts with low co-evolutionary DI scores are filtered out (true interacting sites are depicted in red, and false interacting sites are in black). Step 4: Convergence and energy-guided selection of models—folding and docking EFDOCK-TM simulations enumerating all possible combinations of constraints defined by subsets of predicted contacts are performed, leading to different levels of convergence. A total of 10,000 trajectories and final models are generated per simulation. Representative models are selected among the centres of the five largest families obtained by clustering the 10% lowest-energy models generated by the most-converged simulation. Full size image To assess whether our protocol is effective at enriching evolutionary constraints in inter-chain contacts, we analysed the true positive rate of predicted interactions across the binding interfaces of all characterized TMH homo-oligomer structures as a function of each selection step described in Fig. 3 . As shown in Supplementary Fig. 2 , the rate of true inter-chain contacts increased from an average of 16 to 74% after filtering by LIPS-interacting surfaces and DI score. Except for the tetrameric M2 proton channel of influenza B virus (Inf B) and pentameric phospholamban (PLN), which have too few homologues for reliable detection of residue co-evolution, at least one true interacting site was successfully predicted among the top three strongly co-evolving residue pairs selected for guiding the folding simulations. The high rate of true positive inter-chain contacts in the selected constraints suggests that they may be effective at guiding the de novo structure prediction of TMH oligomers towards the native state. Benchmark EFDOCK-TM was tested on a data set composed of 17 characterized and published TMH homodimer structures and three representative higher-order homo-oligomeric structures determined by high-resolution NMR spectroscopy (Methods). All simulations were performed as in blind predictions: no information from native structures was used and the representative models were selected using the same combination of objective criteria (that is, by all-atom energy and cluster size, Methods). Atomic accuracy prediction of right-handed TM homodimers The experimentally determined interface structures of all six receptors forming right-handed TM homodimers (that is, glycophorin A, Bnip3 and the tyrosine kinase receptors ErbB1, ErbB2, ErbB4 and EphA1) were predicted with atomic accuracy using EFDOCK-TM guided by evolutionary constraints. Consistent with our constraint selection strategy, the best-converged simulations contained a relatively high rate of true inter-chain contacts (64%) and were selected for model accuracy analysis ( Table 1 ; Supplementary Fig. 3 ). For all targets except ErbB1, the largest cluster of low-energy models in our selected simulations was a family of accurate ‘near-native’ models, indicating that a large fraction of the simulations converged towards the native conformation when guided by evolutionary constraints ( Table 1 ; Supplementary Fig. 3 ). The representative selected models displayed atomic accuracy with an average interface Cα-root mean squared deviation (r.m.s.d.) of only 0.83±0.38 Å to the well-defined regions of the NMR structure (Methods; Table 1 ). The backbone structures of the selected representative models in the interacting regions of the homodimers were all superimposable to those of the NMR centre model ( Fig. 4a–f ). Consistent with atomic accuracy predictions, 84% of the native contacts stabilizing the homodimer interfaces were predicted correctly ( Table 1 ). Critical for right-handed homodimer interactions, inter-monomer weak Cα hydrogen bond networks were predicted with atomic accuracy and near-native interfacial side-chain conformations were also consistently observed in these models ( Fig. 5 ; Supplementary Movies 1–6 ). Table 1 Accurate evolutionary-guided de novo prediction of TMH homo-oligomeric structures using EFDOCK-TM. 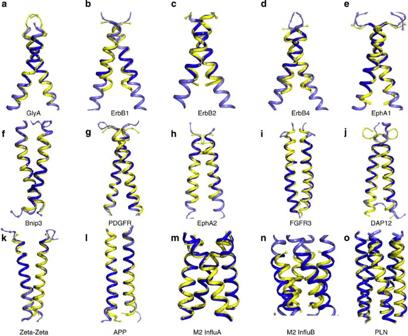Figure 4: Consistent prediction of near-native homo-oligomeric TMH structures. Backbone superposition between the centre NMR model (blue) and the representative EFDOCK-TM model (yellow) of the following receptors: GlyA (a), ErbB1 (b), ErbB2 (c), ErbB4 (d), EphA1 (e), Bnip3 (f), PDGFR (g), EphA2 (h), FGFR3 (i), DAP12 (j), Zeta-zeta (k), APP (l), M2 influA (m), M2 influB (n) and PLN (o). Full size table Figure 4: Consistent prediction of near-native homo-oligomeric TMH structures. Backbone superposition between the centre NMR model (blue) and the representative EFDOCK-TM model (yellow) of the following receptors: GlyA ( a ), ErbB1 ( b ), ErbB2 ( c ), ErbB4 ( d ), EphA1 ( e ), Bnip3 ( f ), PDGFR ( g ), EphA2 ( h ), FGFR3 ( i ), DAP12 ( j ), Zeta-zeta ( k ), APP ( l ), M2 influA ( m ), M2 influB ( n ) and PLN ( o ). 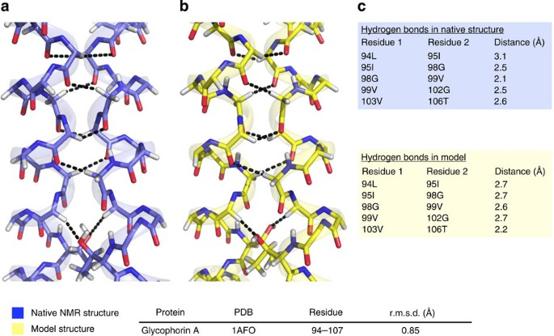Figure 5: Atomic accuracy in right-handed homodimer structure prediction. (a) Backbone representation of glycophorin A centre NMR model (blue). (b) Backbone representation of glycophorin A representative EFDOCK-TM model (yellow). The inter-chain weak hydrogen bond network is highlighted (black dashed lines). The carbon C-alpha root mean square deviation (that is, Cα-r.m.s.d.) of the model over the binding interface region (residues 94–107) is reported at the bottom. (c) Weak hydrogen bond distances in Angstrom are reported for both the native and modelled structures. Full size image Figure 5: Atomic accuracy in right-handed homodimer structure prediction. ( a ) Backbone representation of glycophorin A centre NMR model (blue). ( b ) Backbone representation of glycophorin A representative EFDOCK-TM model (yellow). The inter-chain weak hydrogen bond network is highlighted (black dashed lines). The carbon C-alpha root mean square deviation (that is, Cα-r.m.s.d.) of the model over the binding interface region (residues 94–107) is reported at the bottom. ( c ) Weak hydrogen bond distances in Angstrom are reported for both the native and modelled structures. Full size image Of particular interest is the ErbB2 receptor sequence, which, despite bearing multiple sites for putative weak hydrogen bonds, is not stabilized by such polar networks in the available experimental structure. Modelling predicted inter-chain contacts as direct physical interactions (that is, allowed pairwise Cα distances from 3 to 6 Å as in NMR structure determination, ‘hard potential’; Supplementary Fig. 3a ) allowed large families of accurate models to be generated by EFDOCK-TM (interface Cα-r.m.s.d. of 0.56 Å, Table 1 ; Fig. 4c ). Unlike alternative methods PREDDIMER [30] or CATM [24] , EFDOCK-TM predicted correctly most side-chain conformations and residue contacts at this rather unusual right-handed interface ( Supplementary Movie 3 ). Near-atomic accuracy prediction of left-handed TM dimers Our automated pipeline for constraint selection was also effective at enriching inter-chain contacts at left-handed homodimeric binding interfaces. Except for ErbB3 whose binding interface could not be predicted by LIPS, the most converged simulations were highly enriched in true positive inter-chain contacts (average true positive rate of 83%), thereby generating large clusters of accurate models ( Table 1 ; Supplementary Figs 2 and 3 ). All representative models had an interface r.m.s.d. smaller than 2 Å with an average interface r.m.s.d. of only 1.14±0.45 Å over interface regions spanning an average of 19 amino acids (that is, covering almost the entire TM helix). The backbone structures of our selected representative models were all superimposable to their corresponding NMR structures ( Table 1 ; Fig. 4g–l ) and most buried inter-chain packing interactions and 71% of interfacial residue contacts were predicted correctly ( Fig. 6 ; Supplementary Movies 7–11 ). Of particular interest were DAP12 and zeta–zeta homodimers, which belong to the immune receptor family, participate in the assembly of large hetero-oligomers and are stabilized by several polar interactions. The representative models of zeta–zeta recapitulated all ion pair and hydrogen bond interaction networks with atomic accuracy (interface Cα-r.m.s.d. of only 0.5 Å with up to 100% predicted native contacts for the lowest-energy model; Supplementary Movie 12 ). While the near-native models of DAP12 correctly identified Thr 16 and Asp 20 as hot-spot binding sites at the homodimer interface, they were stabilized by low-energy but non-native polar interaction networks ( Supplementary Movie 9 ). Detailed inspection of the NMR structure revealed that the native conformations of these residues do not form hydrogen bonds according to RosettaMembrane energy function, which may explain why such a configuration was not selected in our simulations. 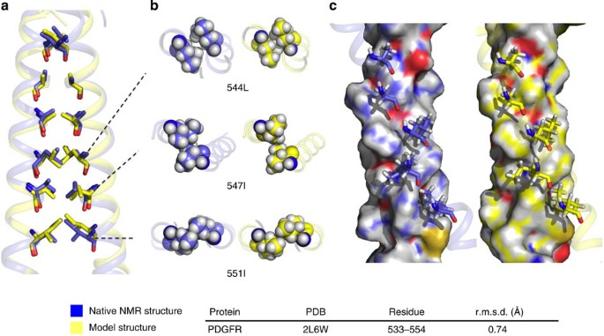Figure 6: Atomic accuracy in left-handed homodimer structure prediction. (a) Superposition of PDGFR centre NMR model (blue) and representative EFDOCK-TM model (yellow) with buried side chains in sticks. (b) Local packing interactions are highlighted for a few buried residues in spheres along the binding interface. (c) Surface representation of the binding interface of one monomer highlighting specific binding grove geometries. The Cα-r.m.s.d. of the model to the native structure over the binding interface region (residues 533–554) is reported at the bottom. Figure 6: Atomic accuracy in left-handed homodimer structure prediction. ( a ) Superposition of PDGFR centre NMR model (blue) and representative EFDOCK-TM model (yellow) with buried side chains in sticks. ( b ) Local packing interactions are highlighted for a few buried residues in spheres along the binding interface. ( c ) Surface representation of the binding interface of one monomer highlighting specific binding grove geometries. The Cα-r.m.s.d. of the model to the native structure over the binding interface region (residues 533–554) is reported at the bottom. Full size image Modelling TM–JM domain improves the TM structure accuracy JM regions (adjacent to TM domains) in SPMRs have been shown to modulate the conformations accessible to the TM domains and to play important roles in propagating signals [19] , [50] . Therefore, we tested the ability of EFDOCK-TM to improve the prediction of the TM region by folding and docking simultaneously TM and JM regions of the characterized Erbb1 and APP TM–JM dimers. For both receptors, simulations were performed with predicted interacting sites in the TM domain and without any constraints in the JM region. Including the JM region significantly enriched the simulations in near-native models for both receptors (that is, additional or higher-ranked clusters of near-native models, Table 1 ; Supplementary Fig. 3 ). Interestingly, APP’s JM domain prevents the GSA motif located near the N-terminal end of the homodimer to interact, which is a low-energy non-native state generated in our simulations of TM homodimers ( Supplementary Fig. 4 ). Higher-order TMH homo-oligomers are predicted accurately We then tested the ability of our approach to predict the structure of higher-order symmetric oligomers, that is, the tetrameric domains of the M2 influenza A and B viroporins and the pentameric domain of PLN. M2 influenza A and PLN were predicted with atomic accuracy (interface r.m.s.d. ≤0.80 Å) ( Table 1 ). Although M2 influenza B and PLN exhibit almost no sequence variation within their homologues, EFDOCK-TM identified the native conformation without constraints. Our representative models of all three targets superimposed well to the experimental structures ( Fig. 4m–o ) with more than 80% of native interhelical packing contacts predicted correctly ( Table 1 ; Supplementary Movies 13 and 14 ). Evolutionary contacts improve TM structure prediction To assess whether evolutionary constraints improve the accuracy of the predictions, identical simulations were performed without constraints. The prediction accuracy of three left-handed and one right-handed dimers (FGFR3, DAP12, APP and ErbB2) markedly increased upon addition of evolutionary constraints (the largest clusters of left-handed models generated without constraints were all non-native; Table 1 ). The number of near-native models among the five largest clusters also largely increased, especially for left-handed targets ( Supplementary Fig. 5 ). Alternative experimental TM structures are well predicted Conformational regulation is a hallmark of membrane receptor function, and several TMH homo-oligomers were characterized in different conformational/functional states. EphA1 TM homodimer structures were solved at low- and high-pH conditions and differ significantly (Cα-r.m.s.d. of 2.7 Å) [51] . The top two lowest-energy clusters among the five largest recapitulated the low- and high-pH structures with Cα-r.m.s.d. of 0.7 and 1.6 Å, respectively ( Supplementary Movie 15 ). Therefore, both conformations of EphA1 would be accurately predicted and selected in a blind prediction. The EGFR TM sequence bears an N- and a C-terminal GAS motif, suggesting two possible binding modes. Indeed, the isolated EGFR TM homodimer was solved in two very different conformations, each stabilized by one of the two motifs (pdb codes: 2M20 and 2M0B; Methods). Experimental and computational studies on the full-length receptor suggest that these conformations represent an active and inactive state occupied by the TM region during receptor signalling [8] , [9] , [21] . Both functionally relevant conformations were accurately predicted by one of the top five clusters of EFDOCK-TM models, with Cα-r.m.s.d. of 1.4 Å (67% native contacts) and 1.0 Å (89% native contacts) ( Supplementary Movies 1, 2 and 16 ). The tetramer M2 proton channel of influenza A virus (M2A) was crystallized in both open and closed states [52] , [53] . Two of the top five clusters including the largest one accurately captured the closed state of M2A, and the open state was predicted by the second and eighth largest clusters with a Cα-r.m.s.d. of 2.90 Å over the TM region, consistent with a lesser-packed and higher-energy open conformation ( Supplementary Fig. 6 ). APP was experimentally observed in two very different conformations, right-handed and left-handed structures which, unlike PREDDIMER [30] , were both predicted correctly by EFDOCK-TM ( Table 1 ). Unlike alternative techniques, our method could also predict multiple experimentally observed conformations of BNIP3 with atomic accuracy ( Table 1 ). EFDOCK-TM outperforms alternative techniques The accuracy of our predictions considerably exceeded that of the method PREDDIMER, which models TM dimer interfaces using ideal helices [30] , especially for left-handed dimers (Cα-r.m.s.d. of 2.86 Å and 17% correctly predicted contacts compared with 1.14 Å and 71% for EFDOCK-TM; Table 1 ). CATM is another technique developed to predict the structure of the GAS motif containing right-handed TM homodimers [24] . Unlike EFDOCK-TM with evolutionary constraints, CATM was not able to predict and select near-native models of the difficult target ErbB2 ( Table 1 ). With an average Cα-r.m.s.d. of only 0.83 Å for right-handed TM dimers, EFDOCK-TM outperformed CATM (Cα-r.m.s.d. of 1.20 Å). EFDOCK-TM outperforms homology-modelling approaches In principle, accurate structural models can be generated from close homologue structures using comparative modelling techniques [31] , [34] . Here we assessed whether available structures are sufficient to derive accurate sequence alignments, templates and constraints to complement the evolutionary-derived EFDOCK-TM approach. Consistent with the very low number of available TM oligomer structures, close structural homologues sharing at least 30% sequence identity and aligning well with target sequences were found for only four receptors (Erbb4, EphA1, influA and influB) in our benchmark ( Supplementary Table 2 ). Consequently, structural accuracy of the threaded templates was low with an average Cα-r.m.s.d. of only 3.4 Å. When relaxed using RosettaMembrane homology-modelling techniques [34] , only four templates could be refined to high accuracy ( Supplementary Table 2 ). While interhelical interactions derived from these templates were of high accuracy for right-handed TM dimers, those derived for left-handed-associated TMs contained only 14% true positive contacts instead of 93% for EFDOCK-TM ( Supplementary Fig. 7 ). When these template-derived contacts were used as constraints in our folding and docking simulations (HFDOCK-TM), right-handed and left-handed models displayed interface r.m.s.d. of 1.2 and 3.8 Å instead of 0.8 and 1.2 Å for EFDOCK-TM models, respectively ( Table 1 ). These results indicate that while associated TM structures may be accurately modelled using constraints from close structural homologues, the scarcity of TMH oligomeric structures currently prevents the wide application of our HFDOCK-TM approach. EFDOCK-TM models are suitable for protein engineering To assess whether EFDOCK-TM models provide structural templates accurate enough for rational protein design applications, we performed native sequence recovery calculations. If native interactions are optimized for stability of the binding interface, then the native sequence should be recapitulated in design calculations. Since the selection of residues in design calculations is very sensitive to the structural environment, native sequence recovery can be used as a strong indication of the accuracy of structural models [34] . To identify which sites are likely optimized for stability, we redesigned the experimental NMR structures and then performed the same calculations using EFDOCK-TM or PREDDIMER models as starting structures. Consistent with the higher accuracy of our EFDOCK-TM models, 86% of the native residues recapitulated using the NMR structures were also recapitulated using the EFDOCK-TM structures compared with only 47% using PREDDIMER models ( Supplementary Fig. 8 ). These results indicate that the EFDOCK-TM models should be accurate enough to guide rational protein design applications, for example, to redesign the binding affinity/specificity of TMH oligomers or to design inhibitors regulating receptor associations and functions. Blind predictions of disease-associated receptor variants The FGFRs and the stem cell growth factor receptor c-Kit are tyrosine kinase receptors binding to the largest family of growth factor ligands, for which a large number of point mutations have been associated with various diseases [1] . A few of these mutations are located in the TM and JM regions of these receptors [1] and are discussed below. Mutations Y372C on the TM–lipid interface and a TM mutation C379R in FGFR1 were found to be strongly associated with osteoglophonic dysplasia, a rare genetic disease characterized by abnormal bone growth. In all five representative FGFR1 models, residues 372 and 379 were predicted to reside on the interacting interface ( Supplementary Fig. 9 ). Two mutations S372C and Y375C were identified in FGFR2 in patients with Beare-Stevenson syndrome, an autosomal-dominant condition characterized by the furrow skin disorder. Y375C is located in the TM region, while S372C belongs to the extracellular JM/TM linker. The largest cluster of FGFR2 models formed a nearly parallel left-handed homodimer with closely packed S372 and Y375 at the interface ( Supplementary Fig. 9 ). The mutation G384R reported in patients with craniosynostosis is located near the middle of the TM region but predicted to be lipid-exposed in our top-ranked models. A single TM mutation G388R in FGFR4 is strongly associated with tumour cell motility. This allele is highly abundant in patients with advanced tumour metastasis. In the two largest clusters of models, G388 formed either weak hydrogen bonds or Van der Waals contacts at the dimer interface ( Supplementary Fig. 9 ). The F522C mutation in the TM domain of c-Kit leads to ligand-independent autophosphorylation and is associated with Mastocytosis. Residue F522 is located at the TM/JM junction of the homodimer and adopt a wide diversity of conformations in our simulations, that is, buried at the binding interface or exposed to the lipid hydrophobic/headgroup interface. Another mutation A533D has been related to diffuse cutaneous mastocytosis. In four among the five top-ranked models, A533 forms contacts across the binding interface at the middle of the TM region of the predicted homodimers ( Supplementary Fig. 9 ). Among the eight mutated sites analysed, six of them were located along the receptor predicted binding interface in the top-ranked models, suggesting a critical role of these positions in controlling protein inter-monomer interaction, associations and function. The two mutation sites predicted to be exposed to the lipids in a fraction of our models were G384R in FGFR2 and F522C in c-Kit. While the G384R mutation may not directly interfere with the interhelical interactions, the presence of an arginine residue in the middle of a TM domain may perturb the membrane insertion of the receptor (due to hydrophobic mismatch that cannot be compensated by lipid deformation when arginine is located at the centre of the lipid membrane) and result in non-functional receptor variants. The F522C mutation may perturb the interhelical interaction or the optimal orientation of the helices in the membrane and affect the regulation of the receptor. SPMR functioning as oligomers represent a large fraction of the human membrane proteome and are involved in crucial functions which when deregulated can lead to severe diseases [1] , [2] , [10] . Experimental evidence indicates that TM and JM domains of many SPMRs participate to signal propagation across the membrane by changing orientation or oligomerization states and by coupling extracellular to cytoplasmic domains [1] , [8] , [9] , [50] . To properly regulate signal transduction, TMHs must be able to switch between states without large energy penalties [1] , [7] . Consequently, TM associations are usually weaker, stabilized by fewer interhelical contacts ( Supplementary Fig. 10 ), conformationally more flexible in single-pass than in multi-pass membrane proteins and very challenging to characterize structurally. In addition, little experimental data on TM–TM or JM–JM interactions is currently available, making the structure prediction of SPMR oligomers also a real challenge. To address this problem, we have developed EFDOCK-TM, a method to predict TMH homo-oligomeric structures from sequence guided by co-evolutionary constraints. By combining TMH-binding surface and residue contact predictions from sequence, we show that sequence co-evolutionary patterns that reflect both intra- and inter-monomer constraints in homo-oligomers can be considerably enriched in inter-chain contacts ( Fig. 3 ; Supplementary Fig. 2 ). When combined with an efficient technique that we implemented to fold and dock TMH oligomers, a small number (2.6 on average) of selected predicted contacts are sufficient to accurately predict the native structure for 21 of 22 TMH homo-oligomers (average Cα-r.m.s.d. of 1.0 Å; Table 1 ; Figs 4 , 5 , 6 ; Supplementary Movies 1–16 ). Our benchmark includes right- and left-handed homodimers and representative higher-order oligomers spanning a wide range of conformations and binding interactions. By contrast, accurate predictions of TMH homo-oligomers so far required numerous experimental constraints [19] , [22] or were restricted to a limited subclass of right-handed homodimers (RHs) stabilized by GXXXG motifs [24] . Left-handed TM dimers (LHs) are particularly challenging to model ( Table 1 ) and the near-atomic accuracy predictions achieved by EFDOCK-TM are unprecedented. While EFDOCK-TM without constraints was able to predict near-native structures of most RHs, the addition of constraints was critical to consistently predict LH structures with high accuracy ( Table 1 ; Supplementary Fig. 3 ). Most RH structures in our benchmark are mainly stabilized by backbone–backbone contacts through weak hydrogen bonds, while LH-binding interfaces often involve greater number but weaker VDW/aromatics contacts between large side chains. Since the latter samples many more conformational degrees of freedom than backbone atoms, side-chain/side-chain contacts may be more difficult to simultaneously optimize. Also, the strong orientational dependencies of hydrogen bond energies make these interactions more specific and may greatly facilitate the search for low-energy native conformations of RH compared with LH structures. Future work will be needed to assess how such differences in chemical interactions between LH and RH structures impact the conformational energy landscape relevant to their function. Discriminating between intra- and inter-chain contacts from co-evolutionary sequence patterns of self-associating proteins is challenging because it requires a systematic and accurate structural interpretation of constraint violations, which can become a daunting task when simulations are performed with a large number of contacts. Interestingly, as shown in Supplementary Fig. 2 , it is the synergistic combination and not each individual constraint selection step alone (EVfold, LIPS and high DI score at predicted binding surfaces) that is effective at enriching for inter-chain contacts. With such a high contact precision, only a small number of constraints (average of 2.6) are needed to select sufficient true positive inter-chain contacts (average of 1.9 per target). Because only very few selected constraints are necessary, accurate prediction may be achievable for a large number of TMH homo-oligomers even when, as observed for many eukaryotic proteins, only relatively few homologue sequences are available (as low as 3 × L with L : modelled protein length). Close structural homologues could be identified for a small number of targets, and the constraints and resulting models derived from these homologue templates (HFDOCK-TM) were of similar accuracy than those generated by EFDOCK-TM ( Table 1 ). However, EFDOCK-TM largely outperformed HFDOCK-TM for most of the targets for which close structural homologues were not available ( Table 1 ). Therefore, while HFDOCK-TM may be a useful approach when close structural homologues can be identified, EFDOCK-TM should be more widely applicable for characterizing the self-associations of eukaryotic membrane receptors. While full-length receptor high-resolution structures have not been characterized to date, current biochemical evidences suggest that TM–TM interactions determined from isolated TM domains and those in full-length receptors are similar [8] , [9] , [19] , [20] , [21] . For example, seminal studies on the EGFR indicate that the TM domain during receptor signalling adopts two conformations (i.e., inactive and active) that are also observed by NMR spectroscopy on the isolated TM region [8] , [9] (Methods). Therefore, these data support a model where TM sequences encode an ensemble of functionally relevant conformations that are ‘selected’ by extramembrane domains and ligands during signalling. Because inter-chain contacts at the TMH-binding interface may have evolved to stabilize multiple conformations [8] , [9] , [16] , [18] , performing simulations using a soft constraint potential allows EFDOCK-TM to populate multiple minima compatible with similar binding surfaces. Alternative conformations may correspond to functionally relevant states of SPMRs as reflected by our ability to predict multiple TM conformations of the EphA1, EGFR, Bnip3 and APP receptors. As demonstrated in previous studies [34] , [54] and in our native sequence recovery calculations ( Supplementary Fig. 8 ), near-atomic structure accuracy, which allows a majority of binding contacts to be accurately predicted ( Table 1 ), is sufficient to design accurate physical interactions. Therefore, engineering TMH inhibitors binding with high affinity and selectivity to receptor-binding surfaces modelled using our method should be feasible. This would extend computed helical anti-membrane protein (CHAMP)-based approaches [1] , [55] to target a large diversity of TMHs for which no structural homologues or specific sequence/structure motifs can be identified. In summary, we have developed a general method that can accurately predict from sequence the structure of a large diversity of TMH homo-oligomers, which to our knowledge is unprecedented. Our approach may prove useful for uncovering the determinants of molecular recognition and regulatory mechanisms of SPMR signalling. Selection of targets for the benchmark data set Single-TM helix homodimers and representative homo-oligomers with solved experimental structure were selected: right-handed (PDB code: 2M20 (ref. 8 ), 2JWA [16] , 2LCX [56] , 2K1K [51] and 2K1L [51] , 1AFO [15] , 2J5D [57] , 2KA1 (ref. 26 ), 2KA2 (ref. 26 ) and 2LZ3 (ref. 58 )), left-handed TM homodimers (PDB code: 2M0B, 2L9U [59] , 2K9Y [28] , 2LZL [27] , 2L34 (ref. 60 ), 2HAC [3] , 2L6W [61] and 2LOH [62] ), tetramers (PDB code: 3LBW M2A closed state [52] , 3BKD M2A open state [53] and 2KIX [63] ) and pentamer (PDB code: 2KYV [64] ). Modelled regions included both residues in the TM and residues in the water–lipid interface regions. The JM region of three targets (amyloid precursor protein, ErbB1 and PLN) was also included in the modelling. The JM regions of ErbB1, APP and PLN were defined between residues 677–690, 686–698 and 1–22, respectively. Blind prediction of disease-related receptor variants Four receptors from the tyrosine kinase family (FGFR1, FGFR2, FGFR4 and c-Kit) with no experimental structures were selected that have multiple reported disease-causing mutational variants in the human population [1] , [65] . Interacting site prediction from protein co-evolution Co-evolution-based contacts were predicted using EVfold [42] , which is based on an inverse covariance matrix-based statistical model. Multiple sequence alignment (MSA) for each candidate protein was performed using HHblits [66] searching against the entire Uniprot database with a range of different E -values. Full-length sequences were used directly as query for small targets (full-length ≤350 amino-acid residues) but were truncated for large targets to allow for optimal alignment of the TM regions. Truncated sequences consisted in the TM region flanked by one conserved extramembrane globular domain on each side of the TM region. Sequences with lower than 50% TM region coverage were filtered out. Then, following the published protocol of the method EVfold [42] , the E -value that generated the largest number of sequence homologues with well-aligned TM region was selected for each target. This procedure ensured that the selected MSAs correspond to the optimal tradeoff between the number of sequences in the alignment and the coverage of the region of interest. To infer inter-residue contacts from sequence covariation, the co-evolution-based direct interaction score DI ij between each pair of residues i and j was calculated using EVfold with default settings ( Supplementary Methods ). All residue pairs were ranked by their co-evolutionary coupling strength and filtered using the following criteria: (1) both residues belong to the TM region; (2) due to the intrinsic symmetry of homo-oligomers, only ‘short-range’ residue pairs separated in sequence by eight positions or less were considered; (3) both residues belong to the helical surface predicted by LIPS [49] to be the least likely lipid-exposed, and the most likely the interacting surface; (4) only residue pairs with strong co-evolutionary signals (that is, DI ij ⩾ 0.1) were selected. For targets with no DI ij ⩾ 0.1, the top three constraints ranked by DI score were used in the simulation ( Supplementary Fig. 3 ). Interacting helical surface and site prediction by LIPS For each target, MSAs were selected using E -values as low as those chosen for EVfold that guaranteed a query sequence coverage of at least 0.5 × L ( L : query protein length). From the selected MSAs, sequences with no gaps within the TM region were extracted and used as input to the method LIPS [49] , which splits a helix into seven overlapping surfaces and predicts interacting TMH surfaces based on residue lipophilicity and sequence entropy. For each target, the surface with the lowest LIPS score was selected as the predicted binding interface. If the two top-ranked LIPS surfaces did not differ by more than 0.5 LIPS score, the surface that had the lowest lipophilicity score (which is the least sensitive to the alignment) was selected. The selected helical surface was applied to filter co-evolutionary constraints identified using EVfold. A set of ‘LIPS’-predicted interacting sites was also derived by selecting the residues with the lowest LIPS score on the predicted interacting surface. To compare and select simulations based on convergence, the number of residues selected by the LIPS score was equal to the number of EVfold constraints for the same target. Since LIPS alone does not provide information on interactions between different residues, loose distance constraints were simply defined between the same residues on each monomer (see below). Co-evolutionary signal analysis at binding interfaces Co-evolutionary DI scores were compared for residue pairs making or not inter-chain contacts along the true or the LIPS-predicted binding interface of all TMH homodimers in the benchmark. Residue pairs were defined as true interacting if the distance between at least one of their respective heavy atoms was smaller or equal to 5 Å in the NMR centre model. To mimic the selection of the helix surface by LIPS, the true binding interface was defined by extrapolating to the entire helix the largest solid angle between the interacting residues and the helix centre axis. For tetramers, the above-mentioned procedure would select the entire helix as the interacting surface so only the subset of residues lying in the centre region of the tetramer, that is, the hexahedron enclosed by the four helical axes, were selected. Residue pairs present at the binding interface were separated into two categories: inter-chain-interacting sites, and inter-chain non-interacting sites. Two different sequence separation thresholds were applied for residue pairs i and j: (1). |i—j|≤8, which corresponds to the short-range window used to select predicted interacting sites; (2) |i—j|≤4, which allows to compare residue pairs forming inter-chain contacts to residue pairs always involved in intra-chain contacts. A paired two-sample T -test was used to evaluate the significance of differences in average DI score and high DI score percentage between the two sets of residue pairs in all targets. The high DI score threshold was defined for each target as the lowest DI score among the top three most strongly co-evolving residue pairs for that target. ErbB3 was not included for the predicted LIPS-binding interface because LIPS predicted a non-native binding surface, which did not bear any true interacting residues. In Fig. 2 panels a and c, the average DI score of both sets of residue pairs for InfluA were substracted by 0.1 to facilitate illustration. The same analysis was extended to a representative set of 103 water-soluble coiled-coils. The 103 coiled-coil structures were selected from the CC+ database ( http://coiledcoils.chm.bris.ac.uk/ccplus/search/ ) by searching coiled-coil homodimers with more than 14 residues, and less than 50% redundancy. DI scores were calculated using EVfold as described above. Coiled-coil binding interface was predicted using MULTICOIL [67] . To analyse the statistical significance of DI score differences between two groups of contacts, a paired two-sample T -test was performed. This test is justified because the sample sizes (that is, number of proteins) of the two groups being compared are identical and there is a one-to-one correspondence between the values in the two samples. Evolutionary-guided structure prediction (EFDOCK-TM) To predict de novo the structure of TMH homo-oligomers, we developed EFDOCK-TM, starting from a protocol to fold and dock symmetric water-soluble oligomers [68] . Simulations typically start from a random symmetric coarse-grained conformation generated by fragment insertion, where torsion angles of randomly selected consecutive three- or nine-residue fragments are replaced by those of protein homologues with known structures. For every 1 in 10 fragment insertions, rigid body backbone movements and docking arrangement perturbations are applied simultaneously to one monomer and cloned to the other monomer. Then, all-atom refinement of the coarse-grained models is performed by sampling side-chain conformational degrees of freedom and applying restrained backbone perturbations. The protocol was modified as follows to increase the efficiency of conformational sampling and the accuracy of the membrane protein structural models: (1) TM regions of each protein predicted using OCTOPUS [69] ( http://topcons.cbr.su.se/index.php?about=octopus ) are inserted into a membrane plane object approximating the lipid membrane prior to fragment insertion. (2) Models are scored using a coarse-grained or all-atom energy function developed for membrane proteins [23] . Unless stated otherwise, predicted interacting sites were implemented as ‘soft’ distance constraints between c-alpha atoms characterized by an equilibrium distance ( d eq ) and s.d. of 6.5 (2.5 Å) for co-evolutionary constraints and 7.0 (4.0 Å) for LIPS constraints. Because they are not based on direct contact information, LIPS constraints are less precise in nature so looser distance constraints were applied. Any distance outside the range defined by d eq ±s.d. is penalized using an harmonic potential. While guiding the simulation towards the native state, ‘soft’ constraints still allow the TMH oligomeric structure to be refined and selected by the physical model underlying RosettaMembrane’s all-atom energy function. For all targets, at least two types of simulations were performed: using all co-evolution constraints, and LIPS constraints. If three or more co-evolutionary constraints were selected for a given target, simulations using all possible randomly selected subsets of constraints (at least two) were also performed. The most converged simulation (that is, generating the least clusters of low-energy models) was selected for model analysis. For each simulation, 10,000 trajectories and models (which guaranteed convergence of the simulations) were generated, and the lowest-energy 10% models were clustered along the TM region using the Rosetta clustering method with a cluster radius of 1.5 Å. As in blind predictions, the representative model selected for each target was the most accurate among the centres of the five most populated clusters. Following another blind prediction selection strategy, the clusters were also ranked by the all-atom energy of the cluster centre. The model for the right-handed alternative conformation of the target APP was selected as one of the top five lowest-energy cluster centres. Structure homology-guided structure prediction (HFDOCK-TM) To predict the structure of TMH homo-oligomers using constraints derived from homologues, we first performed sequence/structure alignments using HHpred [70] to identify the TMH homo-oligomer homologues with known structures, which align best with a target sequence, as described previously [34] . Different target sequence lengths were tried, and query sequences corresponding to the TM region were found to generate the best alignments and were used for all targets. The structural homologue whose sequence aligned best (that is, highest HHpred score and no gap in the aligned TM) with that of each target was selected as the structural template. To assess the accuracy of the alignment and the resulting homology models, the target sequence was threaded onto the homologue structures and relaxed to identify low-energy conformations using the homology-based modelling technique of RosettaMembrane [34] . To extract constraints from these homologues, the closest contact at each helical turn of the binding interface in the homologue structure were selected and implemented as distance constraints in the folding and docking simulations that we defined as HFDOCK-TM. The total number of template-derived constraints in the HFDOCK-TM simulations lay between 4 and 7 for each target. The treatment of constraints and the analysis of the simulations using HFDOCK-TM were identical than with EFDOCK-TM. The accuracy (that is, true positive rate) of the template-derived constraints was very similar when considering a larger set of constraints (that is, top two closest contacts per helical turn at the homologue-binding interface). Assessment of homo-oligomer structure prediction accuracy The r.m.s.d. of the binding interface region was calculated to assess the accuracy of the predictions. The interface region was defined by the residues for which experimental inter-monomeric NMR constraints were obtained (from 9 to 24 residues were selected for each target). The r.m.s.d. was calculated between the representative EFDOCK-TM model and the centre NMR model. All calculations were performed using an open-source python script MATCH ( http://boscoh.com/protein/matchpy.html ). Native contact calculation Native residue–residue contacts were defined if the distance between any of the heavy atoms from two residues on each protein monomer was smaller than 4 Å in the experimental structures. Residue–residue contacts in predicted models were calculated using the same criteria. Comparison with alternative techniques CATM and PREDDIMER The accuracy of published CATM models [24] is reported in Table 1 . PREDDIMER [30] models for all TM dimers in our data set were generated using the webserver: http://model.nmr.ru/preddimer/ . The most accurate among all models output by the server is reported in Table 1 . Accuracy of PREDDIMER and EFDOCK-TM models was analysed using identical criteria. Interhelical contact density comparison in TMH proteins The average number of interhelical contacts per helix in self-associated single-pass TMH protein complexes was calculated using all 20 native structures constituting the benchmark. Residue–residue contact was defined if the distance between two heavy atoms is within a certain threshold. Various distance thresholds were applied (4, 4.5 and 5 Å) for comparison. The same calculation was performed on a representative set of 75 non-redundant multi-pass TM helical domains (sequences identity less than 30%) with resolution better than 3.5 Å from the Protein Data Bank. Native sequence recovery For each target, the NMR structures, EFDOCK-TM and PREDDIMER models were selected and all residues making contacts (between two and three residues per helical turn) at the binding interface were randomized to all 20 amino acids and redesigned to identify the combination that minimizes the energy of the homo-oligomer structures using the design mode of RosettaMembrane as previously described [23] . The percentage of native residues recovered by design at the binding interface was calculated for each starting structure, and the intersection of these native recovered sites between NMR and EFDOCK-TM or PREDDIMER models was reported. Method release Softwares to run and analyse the EFDOCK-TM simulations will be released at the time of publication, and detailed information to run the simulations and reproduce the results is provided in Supplementary Methods . How to cite this article: Wang, Y. & Barth, P. Evolutionary-guided de novo structure prediction of self-associated transmembrane helical proteins with near-atomic accuracy. Nat. Commun. 6:7196 doi: 10.1038/ncomms8196 (2015).